Raman phonon emission in a driven double quantum dot The compound semiconductor gallium–arsenide (GaAs) provides an ultra-clean platform for storing and manipulating quantum information, encoded in the charge or spin states of electrons confined in nanostructures. The absence of inversion symmetry in the zinc-blende crystal structure of GaAs however, results in a strong piezoelectric interaction between lattice acoustic phonons and qubit states with an electric dipole, a potential source of decoherence during charge-sensitive operations. Here we report phonon generation in a GaAs double quantum dot, configured as a single- or two-electron charge qubit, and driven by the application of microwaves via surface gates. In a process that is a microwave analogue of the Raman effect, phonon emission produces population inversion of the two-level system and leads to rapid decoherence of the qubit when the microwave energy exceeds the level splitting. Comparing data with a theoretical model suggests that phonon emission is a sensitive function of the device geometry. Devices based on gallium–arsenide (GaAs) are advantageous for hosting qubits because the electron's small effective mass in this material produces a large level splitting, the lack of valley degeneracy in the band structure simplifies operation, and the clean epitaxial interface used to confine electrons leads to inherently low charge noise [1] , [2] . A potential drawback of GaAs and other group III–V compounds [3] is the presence of nuclear spins in the host lattice, which can rapidly dephase electron spin states [4] . Dynamical-decoupling techniques [5] however, have recently addressed dephasing from nuclei, demonstrating [6] that spin coherence can be preserved for times long enough that it is now important to address alternate decoherence mechanisms such as residual charge noise and processes that incoherently couple electrons to phonons [7] , [8] , either directly [9] , or via the spin orbit interaction [10] , [11] , [12] . In this respect, the piezoelectric nature of GaAs, while advantageous for shuttling electrons long distances [13] , [14] , also opens a channel for enhanced relaxation and dephasing, in particular, for qubit states with a charge dipole [15] , [16] , [17] , [18] , [19] . Such phonon generation mechanisms have recently been examined in the context of readout backaction [19] and compared with transport measurements of InAs nanowires [20] , [21] and graphene [21] . Here we investigate a phonon emission process, distinct from the usual phonon-mediated spontaneous relaxation ( T 1 -type) that leads to the qubit decaying to the ground state. This alternate mechanism additionally limits charge coherence in GaAs and complicates microwave control, even in ideal structures at zero temperature. In a microwave version of the well-known optical technique of Raman spectroscopy, this mechanism provides a means of detecting the phonon spectral density created by the unique nanoscale device geometry. Our experimental results are in qualitative agreement with a theoretical model based on a non-Markovian master equation and we suggest approaches to suppress the electron–phonon coupling, which could further improve coherence times and controllability of these qubit systems. Microwave spectroscopy Our system is a charge qubit with one or two electrons in a double quantum dot, controlled by resonant microwaves [22] , [23] , [24] , which drive Rabi oscillations of the electron between the ground and excited states, as shown schematically in Fig. 1a . In the detuned regime where the microwave energy exceeds the qubit level splitting (see Fig. 1b ), we suggest that this system undergoes driven phonon emission, a process which interrupts coherent oscillations and leads to population inversion, as predicted theoretically [25] , [26] . A micrograph of our double quantum dot device is shown in Fig. 1c , including a proximal rf-quantum point contact [27] (rf-QPC), which is used as a sensor to read out the charge state of the system (see Fig. 1d and Methods). Gate voltages V L and V R control the detuning ε of energy levels between the two dots. For ε >> 0 the ground and excited states of the qubit correspond to localizing the electron mostly in the left (1,0) or right (0,1) dot, respectively, (this is reversed for ε << 0). We apply microwaves with an energy close to the qubit splitting at a certain value of ε , coherently driving between ground and excited states. Under these conditions the readout signal exhibits sidebands that appear as lines in the charge-stability diagram offset either side from the ε =0 transition ( Fig. 2b )). We measure the time-averaged probability P of the electron being in the (0,1) charge configuration, calibrated such that P (0,1)=1 for ε <<0 and P (0,1)=0 for ε >>0. 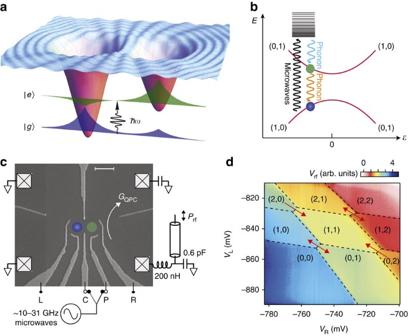Figure 1: Few-electron double quantum dot under microwave excitation. (a) Cartoon of the double dot potential showing a single-electron wavefunction coherently tunnelling between the ground |g› and excited state |e› under microwave excitation. In a microwave analogue of the Raman effect, photon-stimulated emission of phonons (ripples) is modulated by the mode spectrum set by the intra-dot spacing, which for our device is ~280 nm. (b) Energy-level diagram for the single-electron charge qubit showing the stimulated-phonon emission process (light blue) that leads to asymmetric line shapes and population inversion. At a later time, spontaneous emission of a phonon (orange) leads to qubit relaxation. Grey shading depicts virtual states. (c) Micrograph of the double dot device showing surface gates and ohmic contacts to the electron gas (crossed squares). Scale bar, 300 nm. Microwaves are applied to the plunger (P) or centre (C) gate. The conductanceGQPCof a proximal rf-QPC detects the average charge state of the dot and modulates the amount of reflected-rf power,Prf, from a resonant-tank circuit, enabling fast readout (see Methods for details). (d) Charge-stability diagram of the double dot, detected using the rf-QPC. Labels (n,m) denote the number of electrons in the left and right quantum dots, respectively. The demodulated signalVrfis proportional to the QPC conductance and thus the double dot charge configuration. Gate voltagesVLandVRare applied to gates L and R in (c). Red arrows indicate the direction of allowed transitions under resonant-microwave excitation. Figure 1: Few-electron double quantum dot under microwave excitation. ( a ) Cartoon of the double dot potential showing a single-electron wavefunction coherently tunnelling between the ground | g › and excited state | e › under microwave excitation. In a microwave analogue of the Raman effect, photon-stimulated emission of phonons (ripples) is modulated by the mode spectrum set by the intra-dot spacing, which for our device is ~280 nm. ( b ) Energy-level diagram for the single-electron charge qubit showing the stimulated-phonon emission process (light blue) that leads to asymmetric line shapes and population inversion. At a later time, spontaneous emission of a phonon (orange) leads to qubit relaxation. Grey shading depicts virtual states. ( c ) Micrograph of the double dot device showing surface gates and ohmic contacts to the electron gas (crossed squares). Scale bar, 300 nm. Microwaves are applied to the plunger (P) or centre (C) gate. The conductance G QPC of a proximal rf-QPC detects the average charge state of the dot and modulates the amount of reflected-rf power, P rf , from a resonant-tank circuit, enabling fast readout (see Methods for details). ( d ) Charge-stability diagram of the double dot, detected using the rf-QPC. Labels (n,m) denote the number of electrons in the left and right quantum dots, respectively. The demodulated signal V rf is proportional to the QPC conductance and thus the double dot charge configuration. Gate voltages V L and V R are applied to gates L and R in ( c ). Red arrows indicate the direction of allowed transitions under resonant-microwave excitation. 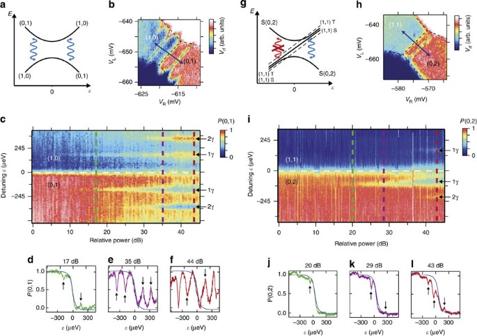Figure 2: Population inversion and asymmetric broadening of microwave spectra. (a) Avoided crossing of the energy levels for the (0,1)–(1,0) transition under microwave excitation. Blue arrows indicate allowed microwave transitions. (b) Charge-stability diagram showing microwave sidebands on either side of the (0,1)–(1,0) transition. The slight broadening of the feature near the transition boundaries is owing to microwave excitation to the leads. (c) Readout probabilityP(0,1) for an electron in the (0,1) state as a function of detuningεand microwave power, where 0 dB is arbitrarily set to a power that yields no effect on the data. Microwave frequencyf=31.8 GHz, applied to gate C. One- and two-photon sidebands (marked 1γ and 2γ) are visible. (d–f), Slices through (c) at different microwave powers, as indicated by the vertical-dashed lines overlaying (c). (g) Energy levels of the two-electron system under microwave excitation. Blue and red lines indicate different rates for microwave driving when the (0,2) singletSis the ground state, verse in (1,1) where the tripletsTare present. (h) Stability diagram at the (0,2)–(1,1) transition with microwaves applied. Sidebands are visible in (0,2) but appear strongly suppressed in (1,1) owing to Pauli spin-blockade. (i) Readout probabilityP(0,2) for an electron in the (0,2) state as a function of detuningεand microwave power. Microwave frequency isf=26.7 GHz, applied to gate P. One- and two-photon sidebands (marked 1γ and 2γ) are visible in (0,2) but are highly suppressed in the (1,1) regime. With increasing power these sidebands asymmetrically broaden on the blue-detuned side closest to∈=0. (j–l), Slices through (i) at positions indicated by the dashed lines in (i). Full size image Figure 2: Population inversion and asymmetric broadening of microwave spectra. ( a ) Avoided crossing of the energy levels for the (0,1)–(1,0) transition under microwave excitation. Blue arrows indicate allowed microwave transitions. ( b ) Charge-stability diagram showing microwave sidebands on either side of the (0,1)–(1,0) transition. The slight broadening of the feature near the transition boundaries is owing to microwave excitation to the leads. ( c ) Readout probability P (0,1) for an electron in the (0,1) state as a function of detuning ε and microwave power, where 0 dB is arbitrarily set to a power that yields no effect on the data. Microwave frequency f =31.8 GHz, applied to gate C. One- and two-photon sidebands (marked 1γ and 2γ) are visible. ( d – f ), Slices through ( c ) at different microwave powers, as indicated by the vertical-dashed lines overlaying ( c ). ( g ) Energy levels of the two-electron system under microwave excitation. Blue and red lines indicate different rates for microwave driving when the (0,2) singlet S is the ground state, verse in (1,1) where the triplets T are present. ( h ) Stability diagram at the (0,2)–(1,1) transition with microwaves applied. Sidebands are visible in (0,2) but appear strongly suppressed in (1,1) owing to Pauli spin-blockade. ( i ) Readout probability P (0,2) for an electron in the (0,2) state as a function of detuning ε and microwave power. Microwave frequency is f =26.7 GHz, applied to gate P. One- and two-photon sidebands (marked 1γ and 2γ) are visible in (0,2) but are highly suppressed in the (1,1) regime. With increasing power these sidebands asymmetrically broaden on the blue-detuned side closest to ∈ =0. ( j – l ), Slices through ( i ) at positions indicated by the dashed lines in ( i ). Full size image Population inversion and spin-dependent transitions Close examination of the microwave sideband lineshape reveals that they are strongly asymmetric and distinct from the characteristic Lorentzian lineshape expected for a driven two-level system. This is seen clearly with increasing microwave power in Fig. 2c , which shows pairs of sidebands corresponding to single- (1γ) and two- (2γ) microwave photon processes, positioned either side of the (1,0)–(0,1) transition. We note that the lineshape of all sidebands is strongly broadened, mostly on the side closest to ε =0, which we refer to as the blue-detuned side, where the microwave photon energy exceeds the qubit splitting. Further, at high powers, we observe population inversion with the amplitude of the microwave sidebands exceeding the saturation value of P (0,1)=0.5 expected for a driven two-level system undergoing Rabi cycles between the ground and excited state. Our device can also be configured to the (2,0)–(1,1) charge transition by adjusting the gate potential to allow two electrons to occupy the double dot (see Fig. 1d ). Under microwave excitation we again observe sidebands that are strongly asymmetric in their lineshape. A key difference in the two-electron case however, is the presence of Pauli-blockade [28] , which leads to spin-dependent transitions when driving resonantly with microwaves [29] . This behaviour is evident in Fig. 2e–h as a strong suppression in the sideband amplitude on the (1,1) side of the transition, where ε >0. We attribute this suppression to the occupation of a triplet state, which cannot tunnel to the (0,2) singlet state under microwave excitation without a spin flip. The maximum height of the suppressed sideband in (1,1) is set by the ratio of singlets to triplets, (1:3 → (0.25 × P (0,2)=0.5), gives P =0.125). We find that this spin-dependent suppression is unchanged for magnetic fields in the range B =0−4T. This field dependence is somewhat in contrast to the recent work by Schreiber et al. , [29] where spin blockade is lifted with microwave excitation, perhaps owing to the presence of a micro-magnet on the surface of their device. The asymmetric lineshape of the sidebands and apparent population inversion is suggestive of the incoherent, Raman-like process described in references [25] , [26] . In this mechanism, a blue-detuned photon drives the qubit transition, accompanied by the emission of a phonon, which carries away the residual energy. The energy (and thus the wavelength) of this phonon is set by the difference between the microwave photon and qubit energies (see Fig. 1b ). Inversion is predicted to occur if the rate of this photon-excited process exceeds the relaxation rate of the qubit. We rule out alternate mechanisms to explain P >0.5, such as an inadvertent-third level, by noting that both sidebands, either side of ε =0, produce the same amount of population inversion. This would imply equal coupling to the third level from both quantum dots, which is highly unlikely for these few-electron devices. Spectroscopic signature of the phononic environment In this Raman picture, the probability for phonon emission is weighted by the density of available modes subject to the boundary conditions of the nanoscale device geometry. In an effort to uncover this geometric fingerprint in the lineshape, a signature of the Raman process, we make use of the high bandwidth of the rf-QPC-charge detector to rapidly average over many data sets so that the sidebands can be observed with high resolution, as shown in Fig. 3a–d for a range of microwave powers. Comparing the averaged data to the Lorentzian lineshape expected for a weakly-driven qubit in the Markovian regime [30] (solid line), it is evident that the blue-detuned region of the sideband shows fine, step-like features [26] in the excited-state probability P (0,1) as a function of detuning. On the ‘red’ side, the data also deviates slightly from the Lorentzian form and exhibits additional structure. Based on a comparison to a detailed-theoretical model [31] , we qualitatively account for these features as arising from the Raman-like process that occurs when the driven qubit is strongly coupled to its phononic environment. 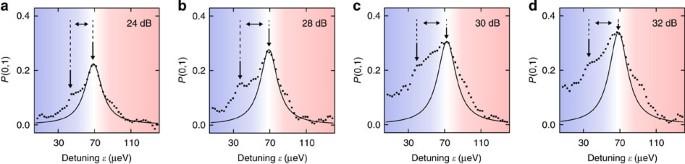Figure 3: Spectroscopic signature of the phononic environment of the double quantum dot. (a–d) Sideband lineshape for weak driving in the one electron configuration, as a function of detuning and for increasing relative powers atf=31.8 GHz (data taken with different tunnel coupling and gate voltages toFig. 2). In the blue-detuned region (ε<~70 μeV), phonon emission results in asymmetric broadening of the sideband and the appearance of step-like features with a spacing (indicated by double arrows) that is set by the distance between the two quantum dots. Extracting this distance from the spacing of the steps gives 280 nm, consistent with the micrograph shown inFig. 1c, see Methods. In the red-detuned region (ε>~70 μeV), the sideband also deviates from the ideal-Lorentzian shape, exhibiting additional skirting features, which we attribute to a renormalization of the qubit levels owing to coupling to the phononic environment. Solid lines are Lorentzian fits to the data using only data points in red region and at the top of the peak. Figure 3: Spectroscopic signature of the phononic environment of the double quantum dot. ( a – d ) Sideband lineshape for weak driving in the one electron configuration, as a function of detuning and for increasing relative powers at f =31.8 GHz (data taken with different tunnel coupling and gate voltages to Fig. 2 ). In the blue-detuned region ( ε <~70 μeV), phonon emission results in asymmetric broadening of the sideband and the appearance of step-like features with a spacing (indicated by double arrows) that is set by the distance between the two quantum dots. Extracting this distance from the spacing of the steps gives 280 nm, consistent with the micrograph shown in Fig. 1c , see Methods. In the red-detuned region (ε>~70 μeV), the sideband also deviates from the ideal-Lorentzian shape, exhibiting additional skirting features, which we attribute to a renormalization of the qubit levels owing to coupling to the phononic environment. Solid lines are Lorentzian fits to the data using only data points in red region and at the top of the peak. Full size image Theoretical model Our model describes the driven system with a master equation in which the Rabi frequency is comparable with the decay rate. To incorporate Raman processes in the weak-driving limit our model does not make the usual assumption of Markovian dynamics [26] , [30] . Taking the Laplace transform of the von Neumann equation gives a series expansion of the dynamical steady state, dependent on the microwave energy detuning, the inter-dot tunnelling rate Δ, the electric dipole Rabi frequency Ω, the microwave-driving frequency ω 0 , the temperature T , and the spectral density, J (ω)=2π∑ q | g q | 2 δ( ω − ω q ), where g q is the device geometry-dependent electron–phonon coupling amplitude, ω q is the phonon frequency and ω is the transition frequency. 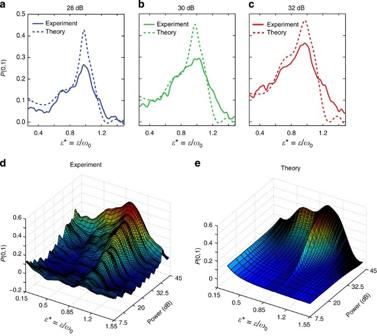Figure 4: Comparison of phononic structure in the theoretical model and experimental data. (a–c), Qualitative comparison between our theoretical model (dashed) and experimental data (solid) for the upper sideband as a function of microwave power (applied to the C-gate).ε* is the dimensionless detuning, normalized by the microwave angular frequencyω0=2π × 32 GHz. (d) Experimental data as a function of detuning showing the evolution of the step-like feature (on the left side of the sideband peak) with microwave power. (e) Theoretical results using parameters for GaAs and independently measured experimental conditions (see Methods). Colouring emphasizes the sideband amplitude. Note that charge noise, when averaged by the rf-QPC, rounds-out the sharper features in the experimental data. Figure 4 highlights the asymmetric lineshape of the sidebands and allows for a qualitative comparison between the experimental data and our theoretical model based on the material properties of GaAs (see Methods for details). Given that the global scaling of the microwave amplitude is the only free parameter in the model, we are unable to quantitatively account for all of the features in the data, particularly in the presence of charge noise. Never-the-less, the clear asymmetry and step feature on the blue side of the sideband can be identified in theory and experiment. Figure 4: Comparison of phononic structure in the theoretical model and experimental data. ( a – c ), Qualitative comparison between our theoretical model (dashed) and experimental data (solid) for the upper sideband as a function of microwave power (applied to the C-gate). ε * is the dimensionless detuning, normalized by the microwave angular frequency ω 0 =2π × 32 GHz. ( d ) Experimental data as a function of detuning showing the evolution of the step-like feature (on the left side of the sideband peak) with microwave power. ( e ) Theoretical results using parameters for GaAs and independently measured experimental conditions (see Methods). Colouring emphasizes the sideband amplitude. Note that charge noise, when averaged by the rf-QPC, rounds-out the sharper features in the experimental data. Full size image With this model in hand, we can now make the case that the Raman-like process indeed accounts for the key features in the data. We rule out photon emission, as the microwave photon lifetime for a dipole of size ~300 nm is a few milliseconds, orders of magnitude longer than that for phonon emission [30] and improbable on the timescale of our experiment. In addition to the population inversion [25] , [26] , the presence of a step-like feature on the blue-detuned side of the resonance is a further signature of resonantly enhanced phonon coupling. The energy of the emitted phonon must be given by the difference between the microwave photon energy and the qubit-excited state (to conserve energy), and when the corresponding wavelength of this phonon is commensurate with the inter-dot separation, the electron–phonon coupling rate is enhanced. The observed spacing of the step-like feature in our data indicates an inter-dot spacing of 280 nm, which is consistent with the geometry of the surface gates shown in Fig. 1c , (see equation 1 and discussion in Methods). Further evidence for the phononic mechanism is given by the apparent shoulder on the red-side of the sideband, which is expected from a renormalization of the qubit detuning and Rabi frequency when the bare electron interacts with the crystal lattice. There are further simplifications in our model that likely account for discrepancies with respect to the position and amplitude of some of the experimental features (in addition to the charge noise mechanism discussed above). These include the anisotropy of the piezoelectric coupling, which we have neglected in our calculations. Further, we have not considered the presence of the surface, which modifies the phononic spectral density. For the present device, where the double dots are located 110 nm below the surface, constructive interference between the double-dot dipole and its image charge couple the electrons to Rayleigh surface acoustic waves. We note that the ability to control the crystallographic orientation of the double dot and its depth from the surface offers a means of suppressing electron–phonon coupling, an advantage of heterostructure devices. Future approaches to suppressing the influence of the phononic environment may include patterning the surface or shaping the gate electrodes to induce phononic band gaps [32] that extend qubit coherence in these systems. Device and experimental setup The double dot is defined electrostatically, 110 nm below the surface of a GaAs/Al 0.3 Ga 0.7 As heterostructure grown using molecular beam epitaxy (electron density 2.4 × 10 15 m −2 , mobility 44 m 2 V −1 s −1 at 20 K). All data is taken at the base electron temperature of a dilution refrigerator, T e ~ 100 mK, with the sample mounted on a custom high-frequency-printed circuit board [33] . Microwave excitation is produced using a room temperature vector source (Agilent 8267D) and fed to the device printed circuit board via coaxial cables that include cryogenic attenuators. Readout is performed using an rf-QPC, proximal to the double dot. An impedance matching tank circuit operating at a frequency of ~500 MHz transforms the high-QPC resistance towards the 50 Ω characteristic impedance of a transmission line enabling the QPC to modulate the amount of reflected-rf power. The change in reflected-rf power is amplified using cryogenic and room temperature amplifiers and demodulated using standard-quadrature mixing techniques to yield a baseband signal V rf proportional to the QPC conductance. For high resolution data ( Figs 3 and 4 ) a high bandwidth digital storage scope is used to perform a large number of trace averages. Theoretical model To compare our theoretical model to the experimental data, we normalize each quantity with respect to the microwave-driving frequency, for example, ω *= ω / ω 0 , where the * indicates dimensionless parameters. In this form we can write: where d *= d ω 0 / c s , with d the inter-dot separation and c s is the transverse speed of sound. where ℏ P is the piezoelectric electron–phonon coupling strength, μ is the mass density, and ω c ≈2π c s / a is a high-frequency cutoff determined by the exponential decay length of the localised electronic wavefunction, a . For GaAs, c s =3,000 ms −1 , ℏ P =1.45 eV nm −1 and μ =5,300 kg m −3 , so P *=0.09. For the driving frequency ω 0 =2π × 32 GHz pertinent to Fig. 4 , we find d *~20. The tunnelling rate Δ*=0.15, and temperature T *= k B T / ω 0 =0.12 are obtained independently from experimental data. We choose , consistent with a ~50 nm. The spectral density in equation (1) exhibits plateaus at ω photon / c s ~(3/2+2 n )π/ d , that is, when the Raman phonon wavelength is commensurate with the interdot spacing. This results in the step-like features in P (0,1) when the detuning matches ω phonon . The first step in P (0,1) occurs at a detuning of 2π × 8 GHz~ ω photon =(3/2)π c s / d (and taking c s =3,000 ms −1 ), we find d ~280–300 nm, consistent with the geometry of the surface gates. How to cite this article: Colless, J. I. et al. Raman phonon emission in a driven double quantum dot. Nat. Commun. 5:3716 doi: 10.1038/ncomms4716 (2014).